Streptococcus agalactiaeclones infecting humans were selected and fixed through the extensive use of tetracycline Streptococcus agalactiae (Group B Streptococcus , GBS) is a commensal of the digestive and genitourinary tracts of humans that emerged as the leading cause of bacterial neonatal infections in Europe and North America during the 1960s. Due to the lack of epidemiological and genomic data, the reasons for this emergence are unknown. Here we show by comparative genome analysis and phylogenetic reconstruction of 229 isolates that the rise of human GBS infections corresponds to the selection and worldwide dissemination of only a few clones. The parallel expansion of the clones is preceded by the insertion of integrative and conjugative elements conferring tetracycline resistance (TcR). Thus, we propose that the use of tetracycline from 1948 onwards led in humans to the complete replacement of a diverse GBS population by only few TcR clones particularly well adapted to their host, causing the observed emergence of GBS diseases in neonates. S treptococcus agalactiae , or Group B streptococcus (GBS) generate considerable neonatal morbidity and mortality worldwide [1] , [2] . In the 1960s, it became the leading cause of neonatal infections in the US and in Europe. The first descriptions of the increase of GBS disease were reported in 1964 as between December 1961 to June 1963 GBS was described as the most frequent cause of neonatal sepsis at the Boston city hospital [3] and in 1965, when Kexel and Schönbohm [4] reported three independent cases of meningitis caused by GBS at the Children’s Clinic of the University of Bonn in Germany. However, in humans S. agalactiae is primarily a commensal of the digestive and urinary tracts, colonizing about 15–30% of healthy adults [1] . 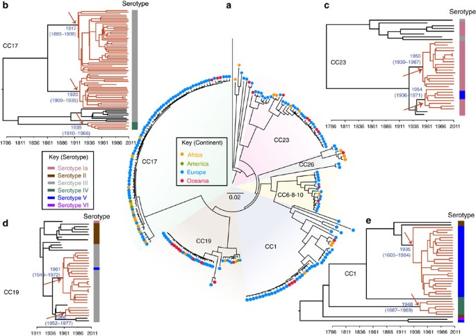Figure 1: Population structure of human GBS is driven by tetracycline resistance acquisition. (a) Whole-genome-based phylogeny of 229 sequenced GBS isolates and strain SS1219 isolated from fish48. Maximum Likelihood (ML) using MEGA was used to infer phylogenetic relationships. The major clonal complexes (CC) 1, 10, 17, 19, 23 and 26 as defined on the GBS MLST web site (http://pubmlst.org/sagalactiae/) correspond to well-defined branches. Isolates are indicated by dots coloured according to their geographical origin. Flanking the whole-genome phylogeny, are four Bayesian maximum clade credibility phylogenies (b–e) based on the non-recombinogenic genome for the GBS CC17 (b), CC23 (c), CC19 (d) and CC1 strains (e). Divergence dates (median estimates with 95% highest posterior density dates in brackets) are provided in blue for the major nodes. Coloured branches relate to the major tetracycline-resistant clones. Arrows indicate the predicted time of insertion of the ICE carrying thetet(M) resistance determinant within the major clones. Capsular serotypes are indicated on the right of each tree according to the indicated colour code. Surprisingly, multi-locus sequence typing (MLST) of GBS isolated from different countries showed that most human carriage and clinical isolates cluster into only five major clonal complexes (CC) (CC1, CC10, CC17, CC19 and CC23) [5] ( Table 1 ). Among those, CC17 strains are considered ‘hypervirulent’ as they are responsible for the vast majority of the meningitis among neonates, and for more than 80% of the late-onset disease cases appearing after 7 days of life [5] , [6] . In contrast, strains responsible for early-onset disease, appearing before the 6th day of life, belong to all five major CCs. A sixth CC, CC26 is common in African countries [7] . In addition to causing disease in humans, GBS is also a veterinary pathogen, causing bovine mastitis [8] . Distinct from human isolates, the majority of bovine isolates belongs to the CC67, a CC for which no human strains have been described [9] . Phylogenetic analysis of 238 isolates of human and bovine origin based on the sequences of 15 genes revealed that CC17 strains represent a homogeneous group of strains of recent origin [9] . The expansion of CC17 strains was suggested to have contributed to the emergence of GBS infections. However, until now, the events responsible for this expansion and the emergence of GBS neonatal infections were unknown. Table 1 Summary of global multi-locus sequence typing studies*. Full size table Here we set out to examine GBS evolution and the rise of neonatal GBS infections. We sequence the genomes of 229 strains isolated between 1953 and 2011 spanning four continents. By combining phylogenetic analyses and the analysis of antibiotic resistance markers, we show that all six human associated CCs have a recent origin and that the observed homogeneity of CC17 strains results from a low rate of recombination relative to the other CCs. Most importantly, we show that the emergence of GBS diseases is associated with the replacement of the bacterial population by a limited number of tetracycline resistant (TcR) clones. Genome-based phylogeny reveals the expansion of a few clones The sequence of 216 GBS genomes of carriage and invasive isolates selected to represent the known diversity of the human GBS population based on MLST studies and of 13 isolates of animal origin was determined. Single-nucleotide polymorphisms (SNPs) were identified by mapping the sequence reads against the genome sequence of a representative ST19 serotype III strain, RBH11. This strain belongs to the dominant CC19 clone that has been shown to display lower levels of polymorphism with strains from other CCs [10] . In total, we identified 40,898 SNPs sites among 1,384,073 interrogated bases unambiguously mapped in the 229 genomes. Using maximum likelihood phylogenetic methods on SNPs in the core chromosome, we determined that 97% of the 216 human isolates clustered into six well-resolved lineages that correspond to the six major human CCs ( Fig. 1a ) as defined by MLST ( Table 1 ). The average polymorphism between lineages is 0.52% (ranging from 0.36 to 0.65%). Strikingly, we observed that within each CC, one or two dominant clones showing limited polymorphisms are present, representing 83% of all isolates. Such a signature is indicative of an evolutionary bottleneck, which has resulted in a recent reduction in population size and expansion of positively selected clones. Figure 1: Population structure of human GBS is driven by tetracycline resistance acquisition. ( a ) Whole-genome-based phylogeny of 229 sequenced GBS isolates and strain SS1219 isolated from fish [48] . Maximum Likelihood (ML) using MEGA was used to infer phylogenetic relationships. The major clonal complexes (CC) 1, 10, 17, 19, 23 and 26 as defined on the GBS MLST web site ( http://pubmlst.org/sagalactiae/ ) correspond to well-defined branches. Isolates are indicated by dots coloured according to their geographical origin. Flanking the whole-genome phylogeny, are four Bayesian maximum clade credibility phylogenies ( b – e ) based on the non-recombinogenic genome for the GBS CC17 ( b ), CC23 ( c ), CC19 ( d ) and CC1 strains ( e ). Divergence dates (median estimates with 95% highest posterior density dates in brackets) are provided in blue for the major nodes. Coloured branches relate to the major tetracycline-resistant clones. Arrows indicate the predicted time of insertion of the ICE carrying the tet (M) resistance determinant within the major clones. Capsular serotypes are indicated on the right of each tree according to the indicated colour code. Full size image GBS CCs except for CC17 show a high rate of recombination Based on the comparison of eight GBS genome sequences, we previously showed that the recombination of large chromosomal segments is a major contributor to the genomic diversification of GBS [10] . Indeed, based on the SNP distribution, here we identified evidence of recombination events encompassing all parts of the core genome ( Supplementary Fig. 1 ), thus distorting the true phylogenetic relationships between GBS lineages. Recombination within each single CC was extensive involving 47% of the genome in CC1, 44% in CC10, 24% in CC19, 42% in CC23 and 19% in CC26 strains but was surprisingly low in CC17, with only 3% ( Fig. 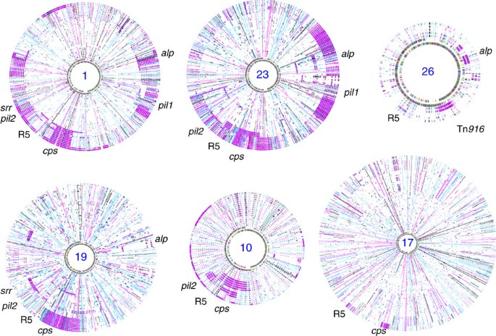Figure 2: Distribution of SNPs and recombination across all GBS isolates from the six major CCs. The maps were generated by using the SyntView software. Isolates were ordered according to the distance from the reference genome depicted at the inner circle. CC numbers are indicated in the centre. Recombined regions compared with the reference genome correspond to regions with a higher density of SNPs indicated by short lines on each circle corresponding to one strain. Around the outside circle are the relative positions of selected antigenic loci. The reference genomes were BG-NI-011 for CC1, DK-NI-008 for CC10, COH1 for CC17, RBH11 for CC19, CCH210801006 for CC23 and Bangui-IP-105 for CC26. 2 and Table 2 ). Most recombination events included genetic determinants for known surface antigens, such as genes encoding the capsular polysaccharide biosynthesis proteins, the major antigenic protein Rib/Alp, the R5 protein, the serine-rich protein and the pili ( Table 2 ), which modulate host–cell interactions [11] . It is therefore likely that immune pressure is a major driving force in the genome diversification of human GBS. Figure 2: Distribution of SNPs and recombination across all GBS isolates from the six major CCs. The maps were generated by using the SyntView software. Isolates were ordered according to the distance from the reference genome depicted at the inner circle. CC numbers are indicated in the centre. Recombined regions compared with the reference genome correspond to regions with a higher density of SNPs indicated by short lines on each circle corresponding to one strain. Around the outside circle are the relative positions of selected antigenic loci. The reference genomes were BG-NI-011 for CC1, DK-NI-008 for CC10, COH1 for CC17, RBH11 for CC19, CCH210801006 for CC23 and Bangui-IP-105 for CC26. Full size image Table 2 Diversity within the six clonal complexes. Full size table Specific GBS clones expanded in the mid-20th century To non-ambiguously reconstruct the evolutionary history of the six GBS lineages, we performed evolutionary studies separately for each CC after mapping the sequencing reads against a representative strain of the CC and filtering out the recombined regions ( Figs 3 and 4 , Supplementary Figs 2–5 , and Table 2 ). This showed that strains of each of the six CCs acquired only a very small number of SNPs, since their respective last common ancestor ranging from 74 to 174 SNPs per Mb. To date the last common ancestor of these clusters and of the nodes corresponding to the major sub-lineages, we performed temporal Bayesian analyses (BEAST) [12] of CC1, CC17, CC19 and CC23 for which the number of isolates and the timespan of isolations provided sufficient posterior support ( Fig. 1b–e ). This analysis estimated that these CCs emerged from a common ancestor within the last 300 years, at a mutation rate of 0.56–0.93 SNP per Mb per year ( Fig. 1b–e ; Table 2 ). These values are in-between the mutation rate predicted for the hypervirulent 027/BI/NAP1 Clostridium difficile variant (0.15–0.53 mutations per year per Mb) [13] and for the globally expanded multidrug-resistant PMEN1 pneumococcus (1.57 mutations per year per Mb) [14] . Nevertheless, the diversification of the six CCs predates by several decades the clinical emergence of GBS neonatal infections that took place in the 1960s [3] ; therefore, the increased incidence of neonatal infections cannot be directly connected to the selection of these clones. Conversely, the majority of the predominant subclones within CC1, CC17, CC19 and CC23, were predicted to have emerged between 1917 and 1966 ( Fig. 1b–e ), a time period corresponding to the observed emergence of neonatal GBS infections. Linear regression of maximum likelihood root-to-tip distances against the year of sampling showed a strong correlation with this data ( Fig. 5 ). This temporal analysis indicates that an evolutionary bottleneck has played a major role in altering the population structure of human GBS within the mid-20th century. 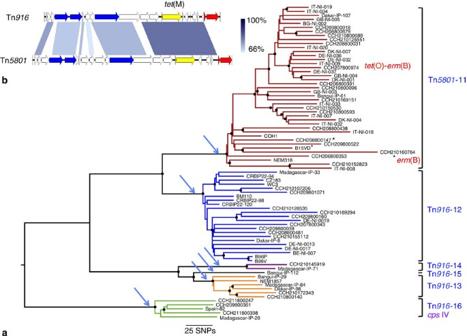Figure 3: Phylogeny of the ‘hypervirulent’ CC17 lineage. (a) ML phylogeny based on the alignment of 3,922 polymorphic positions. Six independent ICE insertions (indicated on the right and by blue arrows) corresponding to six different lineages (indicated by different colours) were identified and are numbered from 11 to 16 (Table 4). A star indicates that Tn5801has been lost by this isolate. Following the loss of Tn5801, strains CCH210160764 and CCH207800974 have acquired unrelated ICE expressingtet(M) anderm(B), andtet(O) anderm(B), respectively. Nodes with >90% bootstrap support are indicated by black dots. (b) Genetic maps and alignment of Tn916and Tn5801. Comparisons were performed by BLASTn. Thetet(M) gene is coloured in yellow, genes encoding type 4 secretion system components are in blue and the integrase and excisionase genes which are not conserved between the two transposons in red. Percentages of identities are shown in blue scale and range between 68 and 98% for thetet(M) region. Figure 3: Phylogeny of the ‘hypervirulent’ CC17 lineage. ( a ) ML phylogeny based on the alignment of 3,922 polymorphic positions. 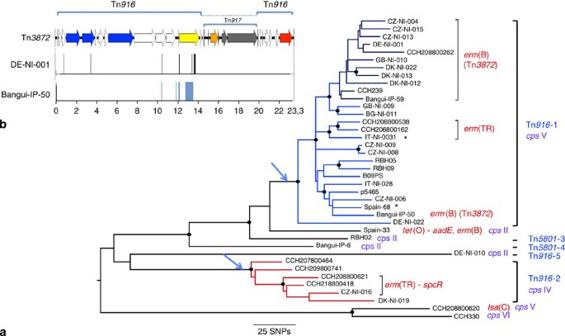Figure 4: Phylogeny of clonal complex CC1. (a) ML phylogeny from the alignment of pseudosequences of the 1,244 polymorphic positions in 914 interrogated kbases. The five independent Tn916or Tn5801insertions are indicated in blue and numbers from 1 to 5 refer to their description inTable 4. The two TcR lineages with more than one isolate are coloured in blue and red. Three sub-lineages have acquired anermresistance gene. Within lineage Tn916-1, 40% of the isolates (12) carry Tn3872(dark-blue branch and strain Bangui-IP-30). The four observed serotypes (cps) II, IV, V and VI are indicated in violet. A star indicates that Tn916has been lost by the isolate. Antibiotic resistance genes other thantet(M) are indicated in red. Nodes with >90% bootstrap support are indicated by black dots. (b) Genetic map of Tn3872. Tn917carrying theerm(B) gene is in grey theerm(B) gene being in orange, Tn916genes are coloured as inFig. 3. The location of 13 out of the 15 SNPs between strain CZ-NI-006 Tn916and strain DE-NI-001 Tn3872, indicated by black bars are located between positions 10,407 and 13,659 (Tn916coordinates) and the 76 SNPs between strain Bangui-IP-50 and strain CZ-NI-006, all located between position 10,407 and 13,497 are in blue. Six independent ICE insertions (indicated on the right and by blue arrows) corresponding to six different lineages (indicated by different colours) were identified and are numbered from 11 to 16 ( Table 4 ). A star indicates that Tn 5801 has been lost by this isolate. Following the loss of Tn 5801 , strains CCH210160764 and CCH207800974 have acquired unrelated ICE expressing tet (M) and erm (B), and tet (O) and erm (B), respectively. Nodes with >90% bootstrap support are indicated by black dots. ( b ) Genetic maps and alignment of Tn 916 and Tn 5801 . Comparisons were performed by BLASTn. The tet (M) gene is coloured in yellow, genes encoding type 4 secretion system components are in blue and the integrase and excisionase genes which are not conserved between the two transposons in red. Percentages of identities are shown in blue scale and range between 68 and 98% for the tet (M) region. Full size image Figure 4: Phylogeny of clonal complex CC1. ( a ) ML phylogeny from the alignment of pseudosequences of the 1,244 polymorphic positions in 914 interrogated kbases. The five independent Tn 916 or Tn 5801 insertions are indicated in blue and numbers from 1 to 5 refer to their description in Table 4 . The two TcR lineages with more than one isolate are coloured in blue and red. Three sub-lineages have acquired an erm resistance gene. Within lineage Tn 916 -1, 40% of the isolates (12) carry Tn 3872 (dark-blue branch and strain Bangui-IP-30). The four observed serotypes ( cps ) II, IV, V and VI are indicated in violet. A star indicates that Tn 916 has been lost by the isolate. Antibiotic resistance genes other than tet (M) are indicated in red. Nodes with >90% bootstrap support are indicated by black dots. ( b ) Genetic map of Tn 3872 . Tn 917 carrying the erm (B) gene is in grey the erm (B) gene being in orange, Tn 916 genes are coloured as in Fig. 3 . The location of 13 out of the 15 SNPs between strain CZ-NI-006 Tn 916 and strain DE-NI-001 Tn 3872 , indicated by black bars are located between positions 10,407 and 13,659 (Tn 916 coordinates) and the 76 SNPs between strain Bangui-IP-50 and strain CZ-NI-006, all located between position 10,407 and 13,497 are in blue. 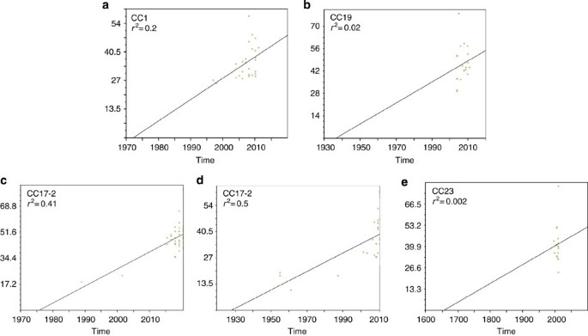Figure 5: Correlation of isolation date with maximum likelihood root-to-tip branch length for the five major TcR lineages calculated with Path-O-Gen. These analyses predict the origin of these clones in agreement with the BEAST analysis except for the CC23 lineage where there was a lack of temporal sampling to support tree root estimates.Xaxis, time in years;Yaxis root-to-tip branch length in SNP per Mb. (a) CC1 lineage Tn916-1; (b) CC19 lineage Tn916-17; (c) CC17 lineage Tn5801-11; (d) CC17 lineage Tn916-12; (e) CC23 lineage Tn5801-23. Full size image Figure 5: Correlation of isolation date with maximum likelihood root-to-tip branch length for the five major TcR lineages calculated with Path-O-Gen. These analyses predict the origin of these clones in agreement with the BEAST analysis except for the CC23 lineage where there was a lack of temporal sampling to support tree root estimates. X axis, time in years; Y axis root-to-tip branch length in SNP per Mb. ( a ) CC1 lineage Tn 916 -1; ( b ) CC19 lineage Tn 916 -17; ( c ) CC17 lineage Tn 5801 -11; ( d ) CC17 lineage Tn 916 -12; ( e ) CC23 lineage Tn 5801 -23. Full size image Human GBS isolates belong mainly to a small number of TcR clones A striking feature of human GBS strains is their high rate (>90%) of TcR, which is predominantly linked with the tet (M) gene encoding an elongation factor G-like protein. Among recent GBS studies, tet (M) was found in 95% of human isolates in Romania [15] , 85% in Kuwait [16] and 91% in Tunisia [17] . In contrast, tet (M)-associated TcR is much less frequent among strains of bovine origin. Specifically, 58% of animal GBS isolates from Portugal were TcR with only 22% expressing tet (M) [18] . Similar observations have been made in France where 39% are TcR and 21% express tet (M) [19] , Estonia, where 22% of strains exhibited varying levels of TcR [20] and in GBS strains isolated from milk in the state of New York where only 14.5% were TcR and 2.5% expressed tet (M) [21] . Furthermore, the tet (M) gene was detected in only 25% of the 51 bovine GBS genome sequences and 10% of the genome of 22 GBS strains isolated from fish that were available at the NCBI database as of 15 May, 2014. These values highlight a very high incidence of tet (M)-associated TcR within human isolates compared with animal GBS. It is known that the use of antibiotics results in a strong positive selection for antibiotic-resistant clones and an overall reduction in bacterial population diversity [22] . To identify a possible link between the population structure of human GBS and antibiotic resistance, we analysed the resistome of the 229 sequenced genomes ( Table 3 ). In agreement with the epidemiological surveys, the most frequent determinants in the 216 human isolates were tet (M) ( n =183, 84%) and tet (O) ( n =10, 5%) both encoding ribosomal protection proteins, and erm (B) ( n =18, 9%) and erm (TR) ( n =12, 5.5%) encoding methylases conferring resistance to macrolides and lincosamides. Other resistance determinants were rare ( Table 3 ). Except for one strain, tet (M) was carried by two related integrative and conjugative elements (ICEs): Tn 916 ( n =111) or Tn 5801 ( n =70) ( Fig. 3b ). In the collection sequenced, Tn 916 and Tn 5801 were found in 23 and 2 different insertion sites, respectively ( Table 4 and Supplementary Table 1 ). Importantly, the expanded clones in all six CCs represent monophyletic lineages sharing the TcR-conferring ICE inserted at the same position ( Table 4 ; Supplementary Table 1 ; Figs 3a and 4a and Supplementary Figs 2–5 ). Moreover, for a given TcR lineage, each transposon shows a maximum of five SNPs supporting a single insertion event for each lineage. These data strongly suggest that the acquisition of ICE harbouring tet (M) has been a landmark event in the expansion of these lineages and in the emergence of the human pathogenic GBS population. Tetracycline was first used in 1948 therefore the subsequent expansion of TcR GBS clones is in agreement with our temporal analysis dating the origin of these clones in the mid-20th century ( Fig. 1b–e ). Interestingly, the major clones include strains from different European and African countries and from Australia, indicating that following their selection, these clones spread globally. Table 3 Distribution of antibiotic resistance genes among the 229 sequenced isolates. Full size table Table 4 Characteristics of clones deriving from Tn 916 and Tn 5801 insertions. Full size table GBS genomes contain a large number of ICEs and other integrative elements. To determine whether the acquisition of other genomic islands has also contributed to the expansion of these clones, we systematically searched for genes specifically acquired by the four major TcR lineages to which the reference genomes belong (CC1 lineage Tn 916 -1, CC17 Tn 5801 -11, CC19 Tn 916 -17 and CC23 Tn 5801 -23). However, we did not find evidence based on the sequenced genomes that such events have taken place. Macrolide resistance contributed to CC1 expansion Tetracycline is not used to treat GBS infections; the most commonly employed antibiotics are ß-lactams, followed by macrolides [23] . Several epidemiological studies reported an increase in the incidence of macrolide resistance in GBS, in particular in strains belonging to the CC1 (ref. 24 ). Indeed, among the 32 isolates of our collection that contained an erm gene, 19 belonged to CC1 (50% of the sequenced CC1 collection) whereas the remaining 13 were sporadically distributed among the other CCs ( Table 3 ). Among the 19 erm -positive CC1 isolates, 17 clustered into three lineages nested into TcR lineages ( Fig. 4a ). In the largest of these three lineages ( n =11 isolates), the erm (B) gene is carried by Tn 917 inserted into Tn 916 leading to Tn 3872 first described in S. pneumoniae [25] . A twelfth isolate, Bangui-IP-50, which belongs to another sub-lineage of the CC1 Tn 916 -1 lineage, also carries a Tn 3872 element. Comparison of the ancestral Tn 916 and the two versions of Tn 3872 showed that the majority of the SNPs (12 out of 15, strain DE-NI-001 and the 76 SNPs, strain Bangui-IP-50) clusters upstream of Tn 917 ( Fig. 4b ). This observation suggests that Tn 917 was inserted in Tn 916 by recombination following the conjugative transfer of two versions of Tn 3872 ; however, we cannot rule out an integration of Tn 3872 following the loss of Tn 916 . In S. agalactiae , Tn 3872 was first identified in four serotype V isolates and one serotype Ia isolate showing similar macro restriction patterns [26] . The erm (B) sequences in these strains are identical to the one present in the major macrolide resistance sub-lineage we have identified, but shows three SNPs over 738 bp in comparison with the Bangui-IP-50 erm (B) gene. Furthermore, the insertion site reported for Tn 3872 is the same as the insertion site of Tn 916 -1. It is therefore likely that the four serotype V isolates carrying Tn 3872 previously described belong to this sub-lineage. These findings show that the erm genes were gained after the acquisition of Tn 916 . Therefore, acquisition of macrolide and lincosamide resistance genes occurred after the selection of the TcR clones, and in the case of the ST1 Tn 916 -1 lineage, has contributed to its clonal expansion. Our analyses indicate that the observed emergence of GBS infections in the 1960s was not due to past under-diagnosis and case reporting of the disease [27] but that it corresponds to a dramatic modification of the human GBS population. Indeed, we show that the human disease-causing and carriage GBS population is dominated be few TcR clones that have spread globally. Tetracycline is a broad-spectrum antibiotic, which was first used clinically in 1948. Subsequently it became widely used, with the first reported case of TcR described in Shigella dysenteriae in Japan in 1953 (ref. 28 ). This timeframe is compatible with the Bayesian estimates that predicted the origin of the GBS TcR clones in four CCs in the mid-20th century ( Fig. 1b–e ) and the identification of three TcR isolates dating back to 1955 within the CC17 clone carrying Tn 916 -12. These three isolates represent the oldest known strains carrying Tn 916 (ref. 29 ). Strikingly, unlike non-CC17 isolates, and despite the larger number of sequenced isolates ( n =79), all CC17 strains belong to clones that have acquired Tn 916 or Tn 5801 ( Fig. 3a and Table 4 ). The absence of a CC17 population naive for these ICEs suggests that CC17 strains were rare before the evolutionary bottleneck exerted by the widespread use of tetracycline. Thus, our data allow us to propose that the acquisition of TcR led to the expansion of hypervirulent CC17 clones that then contributed to the increase of neonatal infections. Due to the broad distribution of resistance in many bacterial species, the use of tetracycline in human health has declined [30] . However, in contrast to what is usually observed for other bacterial species when antibiotic selection pressure decreases, TcR among human GBS remains remarkably stable at the same very high level (>90%). These observations suggest that once inserted in the GBS genome, Tn 916 and Tn 5801 are maintained, as they seem to impose a limited fitness cost to GBS. Indeed, it has been suggested that due to the intricate mechanism of Tn 916 regulation, Tn 916 gene expression likely results in minimizing the biological cost to the host [31] , [32] . It should be noted that the dominance of the tet (M) gene carried by these ICEs is not specific to GBS [31] . Indeed, 133 of 271 Enterococcus faecalis genome sequences available in GenBank as of 15 May, 2014 contain a tet (M) gene, while only 11 contain tet (S) and one tet (O). Furthermore, TcR genes remain the most abundant antibiotic resistance genes identified in human gut microbiota as recently reported [33] . Therefore, the strong selective pressure that tetracycline usage has exerted is more widely observed, but in the case of GBS it has led to the emergence of pathogenic clones. Recombination through the conjugative transfer of large genomic regions has a major role in the diversification of GBS lineages ( Fig. 2 ). In particular, serotype switching due to recombination of the chromosomal region encompassing the capsular biosynthesis locus is the event the most frequently observed. This is also supported by overlaying the capsular serotype distribution onto the Bayesian phylogeny ( Fig. 1b–e ). Indeed, the majority of strains within CC1, CC17, CC19 and CC23 cluster into a dominant capsular serotype ( cps ): CC1/ cps V, CC17/ cps III, CC19/ cps III and CC23/ cps Ia. However, there is a still substantial heterogeneity within CCs relating to capsular serotype. In the case of CC19 and CC23, capsular switching is evident within the major TcR clone. Like the other major CCs examined in this study, isolates belonging to CC17 share a recent origin, however, they differ from the other CCs by a low rate of recombination. Indeed, in this CC, we detected only two recombination events in the early branch leading to the serotype IV ST256 sub-lineage ( Table 2 ). No recombination was identified among CC17 strains, although we have previously shown that, under laboratory conditions, these strains are as permissive to conjugative transfers and recombination as non-CC17 strains [10] . Furthermore, all CC17 strains encode a specific repertoire of surface proteins shown to contribute to increased adherence to intestinal, choroid plexus and microvascular endothelial cells [6] . These observations suggest that CC17 strains colonize a specific habitat leading to genetic isolation. In GBS, the vast majority of Tn 916 and Tn 5801 are inserted in the core genome ( Table 4 ). Therefore, these ICE were acquired by conjugation and tet (M) is likely the major adaptive function not directly associated with genes encoding virulence factors as it has been described in enterococci [34] . However, the expansion of these TcR clones does not explain the concurrent emergence of neonatal infections. We propose as a model that among the selected TcR clones, those with a higher potency to colonize and to disseminate have been selected and have spread across continents replacing less virulent clones. The higher rate of TcR strains and more particularly of the tet (M) gene in human compared with bovine isolates is in support of this hypothesis. A link between antibiotic resistance and increased virulence or transmissibility has been observed for different lineages of opportunistic pathogens leading to the concept of ‘superbugs’ [35] . Examples are the C. difficile clone 027/BI/NAP1, among which two highly virulent lineages expanded following the independent acquisition of resistance to fluoroquinolones [13] , and the epidemic community-acquired methicillin-resistant Staphylococcus aureus clone USA300, which is more virulent than hospital acquired MRSAs, and which emerged from CC8 S. aureus following the acquisition of the methicillin resistance-encoding staphylococcal cassette chromosome mec (SCC mec ) type IV element, and the arginine catabolite mobile element [36] . In USA300, the type I arginine catabolite mobile element is integrated proximal to the SCC mec element, and carries a speG gene which encodes a spermidine acetyl transferase that has been shown to contribute to the dissemination and to the virulence of these strains [37] . Another striking example is the Enterococcus faecium hospital-associated lineages ST17, ST18 and ST78 that are all virulent and resistant to multiple antibiotics including vancomycin [38] , [39] . E. faecium hospital-adapted lineages show a distinct genetic repertoire compared with carriage strains and phylogenomic analysis indicated that they are unrelated to human carrier isolates but they originate from animal strains [39] . However, unique to GBS, the recent evolutionary bottleneck due to the use of tetracycline led to the global replacement of the GBS population colonizing humans. In particular, this bottleneck led to the fixation of the CC17 lineage, which shows a higher virulence in neonates [6] . Therefore, our data strongly suggest that the widespread use of tetracycline has helped drive the emergence of GBS neonatal infections, and created pandemic drug-resistant clones which pose a continued threat to human health. Streptococcus agalactiae (GBS) isolates GBS strains isolated between 1953 and 2011 are listed in Supplementary Table 1 . Their geographical origin, the epidemiological status (early-onset disease; late-onset disease; adult invasive disease, AInv; neonatal invasive disease, NInv; carriage or of animal origin), the year of isolation, the capsular serotype ( cps ) and the sequence type are indicated. Strains were predominantly isolated from Europe (nine countries), Africa (three countries) and Australia. Carriage and invasive strains were selected to reflect the distribution of isolates according to MLST studies ( Table 1 ). CC17 strains were over represented in the collection in an attempt to help characterize the specificity of this hypervirulent lineage. The 12 strains isolated between 1953 and 1961 from the Institut Pasteur bacterial strain collection (CRBIP) belong to CC17, CC19 and CC23. The earliest isolates from the CC1 lineage are from 1997, therefore contributing to lower confidence in dating the origin of this particular lineage ( Fig. 1e ). Thirteen strains are of animal origin. Sequencing, mapping and SNP detection Genomes were sequenced using the Illumina GAIIX or HiSeq2000 sequencing platforms. The read length for each genome is specified in Supplementary Table 1 . The minimal coverage was 75-fold. The sequencing reads were filtered to exclude reads with a quality score of <25 in 10% of the reads and aligned to the reference sequence by using Burrows-Wheeler Aligner [40] . SNP calling was done using SAMtools MPILEUP and varFilter [41] . We excluded SNPs identified in repeated regions, within 100 bp of the contig boundaries from draft reference genome assemblies, or in regions with coverage lower than 40% of the strain’s mean coverage. Reference genomes selected as belonging to the dominant clone of each CC are described in Table 2 . The genome of strain COH1 was completely finished by closing the gaps of the previously determined draft genome sequence [42] . Finishing was performed by Sanger sequencing of PCR products corresponding to gaps and to low-quality regions. The COH1 genome was annotated as previously described [43] . Briefly, coding sequences were defined by combining Genmark predictions with visual inspection of each open-reading frame for the presence of a start codon with an upstream ribosome-binding site and BLASTp similarity searches on Uniref 90, Trembl and Swissprot databases. Function predictions were based on blastp similarity searches and on the analysis of motifs using the Pfam databases ( http://pfam.xfam.org/ ). The five other reference genomes were obtained after ordering the Velvet assembled contigs by using the MAUVE software [44] and the genome of 2603V/R as reference [45] . They were automatically annotated by using the RAST server [46] . De novo assembly and sequence analysis Genome sequences were assembled using the Velvet software [47] with an optimized k -value and a minimal coverage of 10. MLST types were determined by extracting the sequences of the seven genes of the GBS MLST system [5] and comparing them with the known STs from the GBS MLST web server ( http://pubmlst.org/sagalactiae/ ). Serotypes were determined by BLASTn similarity search using as query the nucleotide sequences of the ten cps loci corresponding to the 10 known GBS serotypes. Antibiotic resistance genes were searched by BLASTx search with the protein sequences of 38 resistance genes from Gram-positive bacteria for tetracycline, macrolides, streptomycin, kanamycin, spectinomycin, streptothrycin, lincosamides and chloramphenicol. Genomic islands encoding antibiotic resistance genes were analysed by extracting the sequences surrounding the antibiotic resistance genes. Tn 916 and Tn 5801 insertion sites were determined by analysing the chromosome–transposon junctions ( Table 4 ). Phylogenetic analysis A phylogeny of the 229 GBS isolates sequenced here and the fish isolate SS1219 (ref. 48 ) was constructed by considering nucleotides corresponding to all variable positions located in the core genome for example, in regions present in all isolates. Individual phylogenies of the six CCs were performed after removal of the genomic islands not shared by all isolates, and recombined regions. Automatic detection of recombined regions using the Gubbins software [14] was used to predict genome variation that had arisen by homologous recombination. The ability of this method to robustly predict recombination across the whole population was limited due to the observed genetic diversity of the population, and the corresponding deep branches of the phylogeny. We therefore combined this automatic detection with the visual inspection of variation in each of individual CCs in SyntView [49] viewer ( http://genopole.pasteur.fr/SynTView/flash/Streptococcus_agalactiae ), to identify clusters of SNPs likely to have arisen by recombination. Phylogenetic relationships were inferred using the Maximum Likelihood (ML) method in MEGA5 version 5.10 (ref. 50 ) and the BEAST software v1.7.5 (ref. 51 ). The confidence of the ML tree was estimated using the bootstrap method with 200 bootstrap replications. The trees of the six individual CCs were rooted by using the sequence of an isolate belonging to another CC. The species tree is unrooted. The Bayesian phylogenetic software of BEAST v1.7.5 (ref. 12 ) was used to investigate the temporal evolution of CC1, CC17, CC19 and CC23. The non-recombined variable sites as defined above for each CC was used as markers of ancestral polymorphisms and the year of isolation for each isolate ( Supplementary Table 1 ) was used to calibrate the clock rate. We used the GTR model of nucleotide substitution with four discrete gamma-distributed rate categories and a default gamma prior distribution of 1. To identify the most suitable models, we compared the strict, lognormal relaxed and exponential-relaxed molecular clock models and coalescent constant, exponential growth, expansion growth and Bayesian skyline tree models, using stepping-stone sampling and comparison of log marginal likelihoods [52] , [53] , [54] . Model analyses were conducted in triplicate for 50 million Markov Chain Monte Carlo generations with samples taken every 1,000 generations. Replicate analyses were combined with 10% removed as burn-in using LogCombiner [12] . The Bayesian skyline tree model along with the uncorrelated lognormal relaxed molecular clock to accommodate for rate variation among lineages was preferred. Therefore, final phylogenetic analyses were run in triplicate for 100 million Markov Chain Monte Carlo generations with 10% burn-in using the above parameters. Overall congruency of Bayesian models were observed for all four CCs analysed by BEAST; however, the lack of a wide temporal sampling of strains for CC1 resulted in the lack of an accurate root to accurately define a clock rate, hence the broad confidence values observed in Fig. 1e . Path-O-Gen ( http://tree.bio.ed.ac.uk/software/pathogen/ ) was used to identify a ‘molecular clock’ evolutionary signal as defined by a linear association between the ML root-to-tip branch lengths and year of strain isolation for the five major TcR sub-lineages. This also enabled an alternative method to the Bayesian approach of BEAST to date the expansion event of the five major TcR sub-lineages. ML trees were generated in the sub-lineages: CC1 Tn 916 -1 ( n =26); CC19 Tn 916 -17 ( n =20); CC17 Tn 5801 -11 ( n =41); CC17 Tn 916 -12 ( n =23) and CC23 Tn 5801 -2 ( n =18) from the same recombination-removed SNP alignments used for BEAST analyses. Accession codes: The finished genome of GBS strain COH1 has been deposited in the DDBJ/GenBank/EMBL nucleotide databases with accession code HG939456 . The sequence reads of the 228 GBS Illumina-sequenced genomes have been deposited in the European Nucleotide Archive (ENA) with accession codes ERS039613 to ERS039707 , ERS046905 to ERS046932 , and ERS337437 to ERS337549 (as specified in Supplementary Table 1 ). How to cite this article: Da Cunha, V. et al. Streptococcus agalactiae clones infecting humans were selected and fixed through the extensive use of tetracycline. Nat. Commun. 5:4544 doi: 10.1038/ncomms5544 (2014).